Mechanism of inhibition ofMycobacterium tuberculosisantigen 85 by ebselen The increasing prevalence of drug-resistant tuberculosis highlights the need for identifying new antitubercular drugs that can treat these infections. The antigen 85 (Ag85) complex has emerged as an intriguing mycobacterial drug target due to its central role in synthesizing major components of the inner and outer leaflets of the mycobacterial outer membrane. Here we identify ebselen (EBS) as a potent inhibitor of the Mycobacterium tuberculosis Ag85 complex. Mass spectrometry data show that EBS binds covalently to a cysteine residue (C209) located near the Ag85C active site. The crystal structure of Ag85C in the presence of EBS shows that C209 modification restructures the active site, thereby disrupting the hydrogen-bonded network within the active site that is essential for enzymatic activity. C209 mutations display marked decreases in enzymatic activity. These data suggest that compounds using this mechanism of action will strongly inhibit the Ag85 complex and minimize the selection of drug resistance. According to the World Health Organization, there were 8.7 million new tuberculosis (TB) cases and 1.4 million TB deaths in 2011 (ref. 1 ). The resilience of Mycobacterium tuberculosis ( Mtb ), the bacterium that causes TB, necessitates a treatment regimen of at least 6 months that selects for drug-resistant strains [2] , [3] . In 2011, nearly 20% of cases were multidrug-resistant TB (MDR-TB) and 9% of these MDR-TB cases were also extensively drug-resistant TB. Recently, totally drug-resistant Mtb strains were identified that appear to be untreatable with current antitubercular therapies [4] . Identifying new drug targets and exploiting that information in discovering new antitubercular drugs is of extreme urgency. Many compounds currently in clinical trials target the biosynthesis of the very hydrophobic outer membrane, or mycomembrane, and the arabinogalactan that anchors the inner leaflet of the mycomembrane [5] , [6] , [7] , [8] , [9] , [10] , [11] . This structure is not only important for Mtb viability but is also known to function as a barrier against chemotherapeutic stress by preventing the entry of some antibiotics into the bacterial cell [12] , [13] , [14] . The hydrophobic portion of the mycomembrane is formed by very long, α-branched, β-hydroxy fatty acids called mycolic acids that are either covalently attached to the arabinogalactan forming the mycolylarabinogalactan (mAG) or form the lipophilic tails of extractable glycolipids, such as trehalose dimycolate (TDM), that are located predominantly in the mycomembrane outer leaflet. A variety of other extractable mycolic acid-containing lipids has been identified and shown to impart significant biological effects [15] . The synthesis of TDM and mAG is catalysed by the Mtb -encoded antigen 85 (Ag85) complex, which includes three secreted proteins (Ag85A, Ag85B, Ag85C) with Ag85B being the major Mtb- secreted protein [16] . Belisle et al . [17] established that these enzymes catalyse a transesterification reaction that transfers a mycolic acid from one molecule of trehalose monomycolate (TMM) to another thereby synthesizing TDM ( Supplementary Fig. S1 ) . Other research suggests that Ag85C catalyses the transfer of mycolic acids from TMM to the mAG in vivo [18] . The use of synthetic substrates has confirmed this activity in vitro [19] , [20] , [21] . X-ray crystal structures of all three Ag85 enzymes have been solved. These structures confirmed the highly conserved active site structure, which suggests that all of the Ag85 enzymes use the same mycolic acid donor, TMM, and should allow a single drug to inhibit all three enzymes [22] , [23] , [24] . The X-ray crystal structures also afforded the proposal of a double-displacement catalytic mechanism that proceeds through the formation of an acyl-enzyme intermediate. The rationale for pursuing inhibitors of the Ag85 complex for TB drug development is threefold. As the Ag85 enzymes are secreted, the accessibility of the drug target is increased and common mechanisms of drug resistance such as drug efflux or chemical modification of therapeutics by cytosolic enzymes may be avoided [16] , [25] . Second, current knockout data, particularly the lack of a viable double knockout, suggest that the fibronectin binding protein ( fbp ) genes encoding the Ag85 proteins are synthetically lethal [26] . Therefore, the probability of a strain developing resistance to an Ag85 inhibitory drug would be very low, because mutations promoting resistance in two fbp genes would need to form coincidentally in the same bacterial genome. Finally, modest inhibitors of Ag85 already show decreased viability of Mtb during host infection [27] . This paper describes the efforts that identified ebselen (EBS) as a potent inhibitor of the Ag85 complex and characterized the mechanism of action in vitro and in vivo . Combined with previous data showing a consistent minimum inhibitory concentration (MIC) for both drug-sensitive and MDR-TB [28] , these data indicate that EBS is an intriguing lead for developing new classes of antitubercular drugs to treat MDR-TB. Identification of EBS as a potent Ag85 inhibitor With the knowledge that the Ag85 enzymes possess broad substrate range and can accommodate acyl donors that differ significantly from trehalose, we employ a fluorescent probe that produces a direct measurement of Ag85C enzymatic activity ( Fig. 1a ) [29] . Using resorufin butyrate as the acyl donor at concentrations near the determined K M (62.7 μM) for Ag85C and saturating concentrations of trehalose as the acyl acceptor gives highly reproducible data as indicated by a Z , value determined to be 0.82 (ref. 30 ). Employing this assay for screening of the NIH Clinical Collection (Biofocus) produced multiple hits. Dose-dependent inhibition studies using EBS showed it to be a potent inhibitor with an observed K i value of 63 nM ( Fig. 1b ). 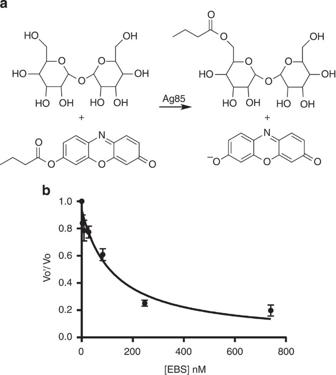Figure 1: Inhibition of Ag85C activity and TDM/mAG production by ebselen. (a) Assay used to measure Ag85C enzymatic activity. The amount of resorufin butyrate converted to resorufin is monitored by measuring fluorescence at 593 nm. (b) Ebselen dose-dependence. Vo′/Vo represents the ratio of the initial velocities of the inhibited reaction (Vo′) and the uninhibited reaction (Vo). Error bars (representing standard deviation or s.d.) are calculated from triplicate reactions. Figure 1: Inhibition of Ag85C activity and TDM/mAG production by ebselen. ( a ) Assay used to measure Ag85C enzymatic activity. The amount of resorufin butyrate converted to resorufin is monitored by measuring fluorescence at 593 nm. ( b ) Ebselen dose-dependence. Vo′/Vo represents the ratio of the initial velocities of the inhibited reaction (Vo′) and the uninhibited reaction (Vo). Error bars (representing standard deviation or s.d.) are calculated from triplicate reactions. Full size image Assays employing authentic substrates ( 14 C-trehalose and cold TMM) not only confirmed the inhibitory activity of EBS on Ag85C but also demonstrated a clear inhibitory effect on Ag85A and Ag85B ( Fig. 2a , Supplementary Fig. S2 ). These experiments unambiguously show that EBS inhibits TDM formation by all three Ag85 enzymes in vitro . 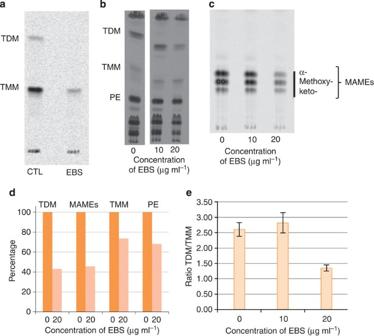Figure 2: Ebselen inhibits mycolyltransferin vitroand inMycobacterium tuberculosis (a) The radiometric mycolyltransferase assay was used to measure the activity of the Ag85C protein in the presence of TMM, [U-14C] trehalose and 0 (CTL: control) or 10 μM EBS. TDM synthesis is completely abolished and the formation of TMM is reduced 70.7% as compared with the control. (b) Effect of EBS treatment for 16 h at 0.5 and 1 × MIC (10 and 20 μg ml−1, respectively) on [14C]-acetate incorporation into TMM, TDM and PE. Total lipids were extracted from bacterial cells as described36. The same volume of each sample was loaded per lane. The TLC was developed in the solvent system (chloroform:methanol:water; 20:4:0.5, v/v) and revealed by autoradiography. PE represents phosphatidylethanolamine. (c) Effect of EBS treatment for 16 h at 0.5 and 1 times the determined MIC value (10 and 20 μg ml−1, respectively) on [14C]-acetate incorporation into cell wall-bound mycolic acids. Cell wall-bound mycolic acid methyl esters (MAMEs) were prepared from delipidated cells36. The same volume of samples was loaded per lane. The TLC was developed three times in the solvent system (n-hexanes:ethyl acetate; 95:5, v/v) and revealed by autoradiography. (d) Effect of EBS treatment for 16 h at 1 × MIC (20 μg ml−1) on [14C]-acetate incorporation into TMM, TDM, PE and cell wall-bound mycolic acids was performed in triplicate. The amount of radioactivity incorporated in the products of interest shown inbandcwas semiquantified using a Phosphorimager and results are expressed as the percentage of the value measured in the untreated cells. PE synthesis was used here as an internal standard to differentiate the specific inhibitory effects of EBS on TDM formation and cell wall-bound mycolic acid transfer from the general and non-specific decrease in [1,2-14C]-acetate incorporation resulting from the loss of metabolic activity in the treated cells. (e) The ratio of TDM/TMM in the untreated control and samples treated with EBS. Error bars (s.d.) are calculated from three independently loaded thin layer chromatography experiments. Figure 2: Ebselen inhibits mycolyltransfer in vitro and in Mycobacterium tuberculosis ( a ) The radiometric mycolyltransferase assay was used to measure the activity of the Ag85C protein in the presence of TMM, [U- 14 C] trehalose and 0 (CTL: control) or 10 μM EBS. TDM synthesis is completely abolished and the formation of TMM is reduced 70.7% as compared with the control. ( b ) Effect of EBS treatment for 16 h at 0.5 and 1 × MIC (10 and 20 μg ml −1 , respectively) on [ 14 C]-acetate incorporation into TMM, TDM and PE. Total lipids were extracted from bacterial cells as described [36] . The same volume of each sample was loaded per lane. The TLC was developed in the solvent system (chloroform:methanol:water; 20:4:0.5, v/v) and revealed by autoradiography. PE represents phosphatidylethanolamine. ( c ) Effect of EBS treatment for 16 h at 0.5 and 1 times the determined MIC value (10 and 20 μg ml −1 , respectively) on [ 14 C]-acetate incorporation into cell wall-bound mycolic acids. Cell wall-bound mycolic acid methyl esters (MAMEs) were prepared from delipidated cells [36] . The same volume of samples was loaded per lane. The TLC was developed three times in the solvent system (n-hexanes:ethyl acetate; 95:5, v/v) and revealed by autoradiography. ( d ) Effect of EBS treatment for 16 h at 1 × MIC (20 μg ml −1 ) on [ 14 C]-acetate incorporation into TMM, TDM, PE and cell wall-bound mycolic acids was performed in triplicate. The amount of radioactivity incorporated in the products of interest shown in b and c was semiquantified using a Phosphorimager and results are expressed as the percentage of the value measured in the untreated cells. PE synthesis was used here as an internal standard to differentiate the specific inhibitory effects of EBS on TDM formation and cell wall-bound mycolic acid transfer from the general and non-specific decrease in [1,2- 14 C]-acetate incorporation resulting from the loss of metabolic activity in the treated cells. ( e ) The ratio of TDM/TMM in the untreated control and samples treated with EBS. Error bars (s.d.) are calculated from three independently loaded thin layer chromatography experiments. Full size image Using a resazurin-based growth assay, the MIC of EBS against Mtb mc 2 6206 was determined to be 20 μg ml −1 , which is identical to that previously published for both drug-sensitive and drug-resistant strains of Mtb [28] . To determine the effects of EBS on Ag85 activity in growing mycobacteria, Mtb mc 2 6206 cultures containing 14 C-labelled acetate were exposed to EBS and the levels of TMM, TDM and mAG-attached mycolates were determined by autoradiography ( Fig. 2b–e ). After a 16-h exposure to EBS at its MIC, EBS exhibits significant inhibition of both TDM and mAG production resulting in a decrease of the TDM to TMM ratio ( Fig. 2e ). TMM synthesis in contrast appeared relatively unaffected. EBS binds covalently to C209 of Ag85C EBS is known to react with thiols to form stable selenenylsulfide bonds [31] . Ag85C possesses a lone cysteine (C209) that is located near the active site at the carboxy-terminal end of the enzyme’s central β-sheet but is not involved in catalysis. To determine if EBS reacts with C209, Ag85C in its native form was incubated with EBS followed by removal of excess EBS by buffer exchange using ultrafiltration. This sample was then subjected to electrospray ionization mass spectrometry (ESI-MS) under denaturing conditions to ensure that any complex observed represented a covalent complex ( Fig. 3a ). The mass difference between the experimental sample and a control sample corresponds to the mass of one EBS molecule, which has an average molecular mass of 274.18 ( Fig. 3b ). These data show conclusively that a single site on Ag85C is covalently modified with EBS. Using the same methodology, EBS is shown to covalently modify Mtb Ag85A and Ag85B at a single site ( Supplementary Figs S3 and S4 ). As an additional control, a similar ESI-MS experiment was carried out using an Ag85C–C209S mutant. In this case, no difference in mass was observed between Ag85–C209S incubated with EBS and Ag85–C209S alone ( Supplementary Fig. S5 ). This strongly supports a hypothesis that the covalent modification of Ag85C by EBS is a consequence of a reaction with C209 following the mechanism proposed in Fig. 3b . 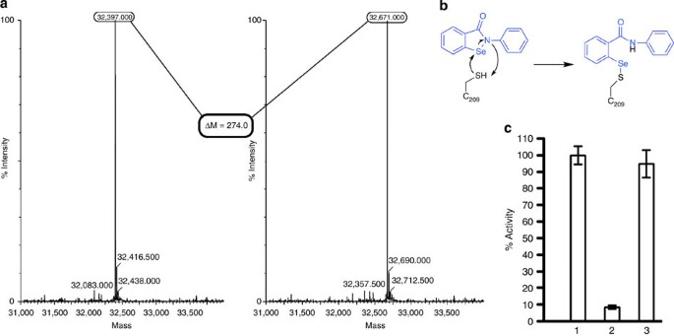Figure 3: Modification of Ag85C by ebselen. (a) Intact mass of Ag85C with and without EBS. On the left, the deconvoluted ESI mass spectrum showing the intact mass of Ag85C. On the right, the deconvoluted ESI mass spectrum showing the intact mass of an Ag85C–EBS covalent complex. (b) Proposed modification of C209 by EBS. (c) EBS forms a reversible covalent complex with Ag85C that inhibits enzyme activity. All excess of EBS has been removed. Activity is normalized to wild-type Ag85C and error bars (s.d.) are calculated from triplicate reactions. Bars 1 and 2 correspond to wild-type enzyme without or with EBS, respectively. Bar 3 is a sample of Ag85C–EBS covalent complex incubated with 1 mM DTT for 24 h. Figure 3: Modification of Ag85C by ebselen. ( a ) Intact mass of Ag85C with and without EBS. On the left, the deconvoluted ESI mass spectrum showing the intact mass of Ag85C. On the right, the deconvoluted ESI mass spectrum showing the intact mass of an Ag85C–EBS covalent complex. ( b ) Proposed modification of C209 by EBS. ( c ) EBS forms a reversible covalent complex with Ag85C that inhibits enzyme activity. All excess of EBS has been removed. Activity is normalized to wild-type Ag85C and error bars (s.d.) are calculated from triplicate reactions. Bars 1 and 2 correspond to wild-type enzyme without or with EBS, respectively. Bar 3 is a sample of Ag85C–EBS covalent complex incubated with 1 mM DTT for 24 h. Full size image To further strengthen this hypothesis, peptide mass fingerprinting experiments using the EBS-modified Ag85C were performed. Both Ag85C as a control and the Ag85C–EBS complex were digested with sequencing-grade trypsin (Promega). Matrix-assisted laser desorption/ionization mass spectrometry analysis of tryptic peptides from Ag85C–EBS revealed that peptides containing C209 exhibit a shift in mass near 274 atomic mass units, which corresponds to the attachment of one EBS molecule ( Supplementary Table S1 ). The observed masses from the Ag85C tryptic peptides that do not contain residue C209 matched those expected from the protein sequence. Together, these data suggest that residue C209 of Ag85C and the analogous C211 of Ag85A and 85B are covalently modified by EBS. As the covalent adduct is a product of C209 oxidation by EBS, covalent complex formation should be reversible using dithiothreitol (DTT). We assessed this by reacting an Ag85C–EBS covalent complex with DTT and subjecting that reaction to ESI-MS. Mass spectrometry data clearly exhibit a decrease in mass concomitant with the loss of one molecule of EBS, thereby exhibiting the reversibility of the covalent modification of Ag85C by EBS under reducing conditions ( Supplementary Fig. S6 ). This suggests that the inhibitory effects imparted by EBS likely occur away from the reducing environment of the mycobacterial cytoplasm. The periplasmic space and extracellular environment are both oxidizing, particularly during late stages of infection when mycobacterial growth is extracellular. C209 modified by EBS leads to a significant loss in activity To assess the effect of C209 modification by EBS on the enzymatic activity of Ag85C, both Ag85C and Ag85C–EBS were assayed using the resorufin butyrate assay under identical conditions ( Fig. 3c ). Prior to performing the assay, the Ag85C–EBS complex was subjected to ultrafiltration to remove excess EBS so the only EBS present in the sample was covalently attached to Ag85C. The Ag85C–EBS complex exhibits almost no enzymatic activity when compared with both the wild-type enzyme and a negative control assay lacking Ag85C. These data show that the covalent modification of C209 with an equimolar concentration of EBS leads to an enzyme with less than 7% activity of the Ag85C enzyme. To determine if reducing the selenenylsulphide bond and thereby reversing covalent modification of C209 by EBS rescues enzymatic activity, an Ag85C–EBS complex already shown to lack enzymatic activity was incubated for 24 h in a solution containing 1 mM DTT and then tested for enzymatic activity. These experiments show that Ag85C recovers wild-type level enzymatic activity when the selenenylsulphide bond is reduced ( Fig. 3c ). As inactivation of the enzyme through modification of C209 with EBS is so pronounced, we pursued experiments that would determine if inhibition is specific to EBS modification or if any modification of C209 eliminates enzyme activity. To this end, Ag85C was modified with iodoacetamide (IAA), which is an alkylating reagent commonly used to identify thiols in biomolecules. Subsequent peptide mass fingerprinting of tryptic peptides resulting from this reaction revealed a mass shift of 57.0 in the tryptic Ag85C peptides containing C209, which corresponds to covalent modification by IAA ( Supplementary Table S1 ). Similar to the Ag85C–EBS complex, the IAA-modified enzyme again exhibits almost no enzymatic activity ( Supplementary Fig. S7 ). However, complete inhibition of Ag85C by EBS is much more efficient than inhibition by IAA ( Supplementary Fig. S8 ). Using EBS at 5 μM concentration, inhibition requires less than 5 min of incubation in vitro , but using a 51.2 mM concentration of IAA in an identical reaction shows a 60% reduction of activity after 1 h and an 80% decrease after an overnight incubation with Ag85C. Therefore, covalent modification of C209 leads to a significant decrease in Ag85C activity and this inhibition appears to be independent of the covalent modifier. C209 mutants exhibit a nearly complete loss of activity A BLAST search using the Ag85C sequence from Mtb strain H37Rv and a subsequent multiple sequence alignment comparing 564 deposited mycobacterial Ag85 sequences and related proteins was performed ( Fig. 4a ). The residue corresponding to C209 in Mtb Ag85C is present in 480 (85%) of the Ag85 enzymes while a serine residue is observed in 76 of these (13%) suggesting that an Ag85C–C209S mutant or other mutation may possess near wild-type enzymatic activity. 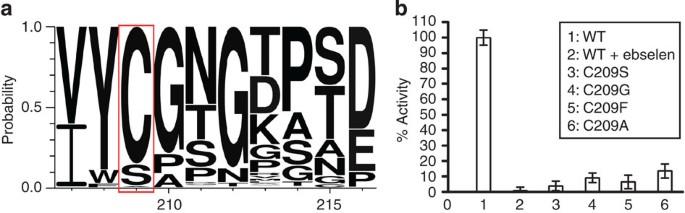Figure 4: Potential mutations of C209 residue on the Ag85 and effect on the enzymatic activity. (a) Sequence logo of mycobacterial Ag85. The logo is from 564 aligned Ag85 sequences. Thex-axis represents the residue number based on that ofMtbAg85C. (b) Mutating C209 inactivates Ag85C. Bars 1 and 2 are wild-type Ag85C without and with EBS (in excess), respectively. Bars 3–5 are single-nucleotide mutants of C209. Bar 6 is a double-nucleotide mutant of C209. Activity is normalized to wild-type Ag85C and error bars (s.d.) are calculated from triplicate reactions. Figure 4: Potential mutations of C209 residue on the Ag85 and effect on the enzymatic activity. ( a ) Sequence logo of mycobacterial Ag85. The logo is from 564 aligned Ag85 sequences. The x -axis represents the residue number based on that of Mtb Ag85C. ( b ) Mutating C209 inactivates Ag85C. Bars 1 and 2 are wild-type Ag85C without and with EBS (in excess), respectively. Bars 3–5 are single-nucleotide mutants of C209. Bar 6 is a double-nucleotide mutant of C209. Activity is normalized to wild-type Ag85C and error bars (s.d.) are calculated from triplicate reactions. Full size image To assess the activity of C209 mutants, the most conservative single-nucleotide polymorphisms of the C209 codon as well as a possible double-nucleotide missense mutant were made and subjected to enzymatic assays. Specifically, the single-nucleotide mutants that encode Ag85C–C209S, Ag85C-C209F and Ag85C-C209G, as well as the two-nucleotide mutant encoding Ag85C-C209A were tested. Each exhibited either a complete loss of enzymatic activity or a profound decrease to less than 10% of wild-type activity ( Fig. 4b ). This suggests that replacing C209 with either small or large hydrophobic side chains leads to an inactive enzyme. EBS alters the Ag85C active site structure All three Ag85 enzymes exhibit an α/β hydrolase fold and a conserved catalytic triad (S124, E228 and H260 in Ag85C) [23] . The hydrogen-bonded network connecting the residues of the catalytic triad imparts a strained kink in helix α9 that harbours E228 ( Supplementary Fig. S9 ). Additionally, helix α9 forms one side of a hydrophobic cleft that is proposed to accommodate a portion of the mycolic acid when bound within the active site. Covalent modification of S124 with a serine protease inhibitor disrupts the hydrogen-bonded network formed by the catalytic triad and allows the relaxation of the strained kink in helix α9 (ref. 23 ). X-ray crystallography experiments were performed to define the structural effects of C209 modification that lead to enzyme inactivation. Ag85C crystallized in the presence of excess EBS was solved to 1.35 Å resolution ( Table 1 , PDB accession code 4MQM ). Although the mass spectrometry data unambiguously demonstrate that EBS forms a covalent bond with C209, and 2Fo-Fc density representing C209 is clearly visible from the diffraction data, density representing EBS or the loop that connects C209 with helix α9 (residues 211–221) is lacking ( Fig. 5 ). For clarity, this newly described structure will be referred to as the Ag85C–EBS structure. Intriguingly, the Ag85C–EBS structure is isomorphous with the Ag85C-mercury co-crystals used to solve the first Ag85C structure. In the Ag85C-mercury crystals, residue C209 was covalently modified with mercury [23] . Table 1 Data collection and refinement statistics. 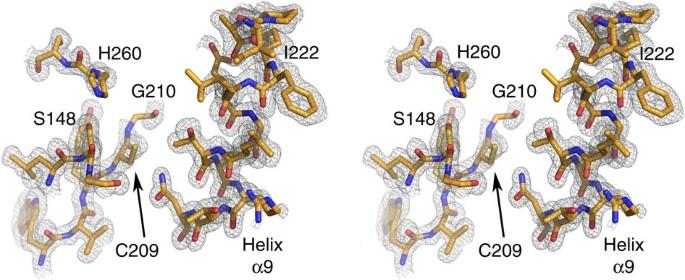Figure 5: Disorder near the modified C209 residue. Shown is a stereo view of the 2Fo-Fc map (blue) contoured at 1σfor the region encompassing C209 of the Ag85C–EBS structure. Bonds for all modelled atoms in the Ag85C–EBS (PDB accession code 4MQM) structure representing the loop region encompassing residues 206–235, as well as H260-S261 and 147–149 are shown and coloured by CPK with carbon atom coloured gold. No density representing the residues T212-N221 is observed suggesting significant flexibility. Density for the H260 side chain is incomplete suggesting moderate disorder. This contrasts with every other Ag85 structure, where the H260 conformation is well ordered by hydrogen bonding with either S124 or S148. The large U-shaped pocket immediately above C209 represents the most likely location of EBS. Full size table Figure 5: Disorder near the modified C209 residue. Shown is a stereo view of the 2Fo-Fc map (blue) contoured at 1 σ for the region encompassing C209 of the Ag85C–EBS structure. Bonds for all modelled atoms in the Ag85C–EBS (PDB accession code 4MQM) structure representing the loop region encompassing residues 206–235, as well as H260-S261 and 147–149 are shown and coloured by CPK with carbon atom coloured gold. No density representing the residues T212-N221 is observed suggesting significant flexibility. Density for the H260 side chain is incomplete suggesting moderate disorder. This contrasts with every other Ag85 structure, where the H260 conformation is well ordered by hydrogen bonding with either S124 or S148. The large U-shaped pocket immediately above C209 represents the most likely location of EBS. Full size image Superimposing the Ag85C–EBS structure with the native Ag85C structure (PDB accession code 1DQZ ) gives a low r.m.s. displacement of 0.53 Å for all Cα atoms indicating that the structures are quite similar over the majority of the polypeptide chain. However, a change in structure is observed near C209 and this propagates structural changes to a portion of the enzyme-active site. In the native Ag85C structure, the C209 side chain abuts helix α9 at the exact position where the helix is kinked ( Supplementary Fig. S9 ). The region enveloping the C209 side chain is hydrophobic in nature and van der Waals interactions predominate between the C209 side chain and helix α9 at the peptide bond between residues T231 and L232. The side chain of C209 does not form specific hydrogen bonds or other polar interactions with any atoms. The Ag85C–EBS structure shows that the kink in helix α9 has relaxed to a straight helical form reminiscent of that observed for the Ag85C–DEP structure (PDB accession code 1DQY ). Indeed, the r.m.s. displacement for the Cα atoms when superimposing the DEP and EBS-modified structures is only 0.44 Å, which shows that the DEP and EBS-modified structures are more similar to each other than either is to the native structure. The primary difference observed in the Ag85C–EBS structure when compared with Ag85C–DEP is an exaggerated shift of helix α9. It is possible that the EBS modification of C209 promotes this conformational change through steric repulsion between the modified residue and the peptide bond between residues T231 and L232 of helix α9 ( Fig. 6 ). These residues have shifted 3.0 Å further away from C209 and when combined with helix α9 straightening, the Cα position for residue E228 has shifted 6.1 Å with respect to the native Ag85C structure, which disrupts the hydrogen bond between catalytic triad residues E228 and H260. This promotes disorder in the H260 side chain and likely decreases its efficiency as a general base to activate the S124 nucleophile. Specifically, H260 Cγ displays a B-factor of 36.4 Å 2 in the Ag85C–EBS structure, but has an average of 14.7 Å 2 in the other available Ag85C structures. Because the C209F mutation and IAA modification both effectively increase the relative size of the side chain at position 209, a similar structural change to that observed in the Ag85C–EBS structure is likely responsible for decreasing the enzymatic activity in those enzymes. 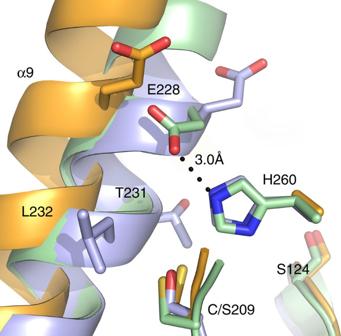Figure 6: Modification at Ag85C residue 209 disrupts the active site structure. The catalytic triads for Ag85C–EBS (orange), Ag85C–C209S (blue) and Ag85C–DEP (green) are shown. Only the Ag85C–DEP structure possesses interactions between any of the catalytic triad. The dashed bond indicates the hydrogen bond between E228 and H260 in the Ag85C–DEP structure. Note that in the native form of the enzyme (not shown), H260 is also hydrogen bonded to S124. Most of the side chain of H260 in the Ag85C–EBS structure is disordered with only the β carbon of the side chain is observed. Figure 6: Modification at Ag85C residue 209 disrupts the active site structure. The catalytic triads for Ag85C–EBS (orange), Ag85C–C209S (blue) and Ag85C–DEP (green) are shown. Only the Ag85C–DEP structure possesses interactions between any of the catalytic triad. The dashed bond indicates the hydrogen bond between E228 and H260 in the Ag85C–DEP structure. Note that in the native form of the enzyme (not shown), H260 is also hydrogen bonded to S124. Most of the side chain of H260 in the Ag85C–EBS structure is disordered with only the β carbon of the side chain is observed. Full size image However, it was unclear if the same structural change is occurring in the other C209 mutants with smaller hydrophobic or polar side chains. The structure of Ag85C–C209S (PDB accession code 4MQL ) was solved to determine if this mutation produces structural changes in the active site similar to that observed in the Ag85C–EBS structure. Indeed, the X-ray crystal structure of an Ag85C–C209S mutant shows that helix α9 straightens in response to this change at position 209, but the active site structure more closely resembles that of the Ag85C–DEP structure. However, like the Ag85C–EBS structure, the hydrogen-bonded network of the Ag85C–C209S catalytic triad is completely disrupted and the structure of residues 210–221 adopts a different conformation compared with the native form of the enzyme. This suggests that the lack of Ag85C–C209S enzymatic activity parallels that of the EBS-inactivated enzyme. Since the first demonstration of enzymatic activity, the Ag85 complex has been considered by many to be an intriguing target for the development of new TB therapeutics [17] . A variety of assays that measure the activity of the Ag85 complex have been developed to afford efficient screening and lead characterization. The radiometric assay developed by Belisle et al . [17] was used to suggest the mycolyltransferase activity but is not amenable to high-throughput screening of compound libraries. Two enzyme-coupled assays developed in 2009 have the potential for use in a high-throughput format [32] , [33] ; but problems with TMM solubility and assay precision have limited their application. In spite of the shortcomings, the assay described by Boucau et al . [33] was used to identify EBS as an inhibitor of Ag85C, but characterizing the inhibitory mechanism was not pursued until a more robust assay was developed [33] , [34] . To this end, the resorufin butyrate assay was developed and used to confirm Ag85C inhibition by EBS and to define the mechanism of action. From the chemical structure of EBS, the possible mechanism of Ag85 inhibition was initially unclear, as it does not structurally mimic substrates, transition states or products. Indeed there are only three heteroatoms in EBS that would promote specific bonding interactions with the enzyme-active site to promote specific Ag85 binding and inhibition. The best hypothesis was that the reactive selenenyl amide moiety of EBS promotes covalent modification of Ag85. Specifically, researchers have exhibited the ability of selenium-containing compounds to label thiols in biological molecules [31] . Xu et al . [31] demonstrated that the thiol moiety of cysteine residues in proteins could form a new selenenylsulphide bond in a highly selective manner that is reversible with reductants such as DTT. Combined with this chemoselectivity and the fact that Ag85C contains only one cysteine residue, the described ESI- and Matrix-assisted laser desorption/ionization mass spectrometry data show conclusively that residue C209 of Ag85C is modified by EBS through the formation of a stable selenenylsulphide bond. The Ag85A and Ag85B ESI-MS data also show covalent modification at a single site. As this cysteine is conserved in all three Mtb -encoded Ag85 enzymes and the only two remaining cysteine residues in Ag85A and Ag85B form a disulphide bond, it is expected that EBS modifies each Ag85 enzyme in the same manner. The selenium atom of EBS is reactive towards any thiol functional group so it is important to determine if EBS inhibits mycobacterial growth by specifically targeting the Ag85 complex or by targeting other enzymes. Published studies have shown that EBS inhibits growth of Helicobacter pylori and suggest this phenotype is a consequence of EBS inhibition of thioredoxin reductase through the formation of a covalent complex with active site cysteine residues [28] . The authors attribute this antibacterial activity of EBS to the lack of glutathione production in Helicobacter and suggest that a similar inhibitory mechanism occurs in Mtb . However, this is unlikely to be the case. Although Mtb does not synthesize glutathione, it produces significant amounts of mycothiol, which possesses analogous function to glutathione [35] . Because of the presence of mycothiol in the mycobacterial cytoplasm and its roles in redox homoeostasis and detoxification, it is unlikely that the primary EBS target in Mtb is located in the cytoplasm. In contrast, formation and stability of a selenenylsulphide bond between EBS and secreted proteins such as those of the Ag85 complex is unlikely to be affected by mycothiol production in the mycobacterial cytoplasm. The culture-based studies that monitored the production of mAG-attached mycolic acids and TDM production support the Ag85 complex as the primary target. These experiments show that the EBS MIC and the concentration of EBS necessary for potent inhibition of Ag85 activity correlate, whereas obviously weaker inhibition of TDM or mAG production is observed at a concentration half that of the MIC. Additionally, the TDM to TMM ratio decreased significantly under these conditions, further suggesting that applying EBS inhibits TDM production but not TMM production. This apparent lack of effect by EBS addition on TMM formation in whole cells is expected, as the intracytoplasmic biosynthesis of TMM is thought to occur prior to the translocation of TMM to the periplasmic space and is most likely independent of the Ag85 complex [36] . Although C209 does not have any role in the catalytic reaction performed by Ag85C, the modification of C209 by EBS clearly affects the ability of Ag85C to catalyse an acyl transfer reaction. To better understand the mechanism of inhibition, X-ray crystal structures of Ag85C in the presence of EBS (PDB accession code 4MQM ) and the Ag85C–C209S mutant (PDB accession code 4MQL ) were solved and compared with previously published Ag85 crystal structures ( Supplementary Fig. S10 ) [20] , [22] , [23] , [24] , [37] . Of the comparable eight X-ray crystal structures of the Ag85 enzymes, five possess a structure where the residues of the catalytic triad (S124, E228 and H260) form a hydrogen-bonded network consistent with an active enzyme and the side chain of C209 (or C211 of Ag85A and Ag85B) is interacting with the kinked region of helix α9 (PDB accession codes 3HRH , 1SFR , 1VA5 , 1DQZ and 1F0N ). Of the remaining three structures, all of which exhibit relaxation of helix α9, none possess significant enzymatic activity. Although the Ag85C–DEP complex is inactive because S124 of the catalytic triad is covalently modified by a serine protease inhibitor, the inactivity of the Ag85C–EBS complex and Ag85C–C209S appears to derive solely from the change in active site structure due to modification at position 209. The hypothesis that C209, and the analogous C211 of Ag85A and Ag85B, is essential for maintaining the appropriate structure of the enzyme-active site is reflected in the decreased enzymatic activity observed in C209 mutants of Ag85C. Single-nucleotide changes at position C209 result in mutants that exhibit less than 10% of the wild-type enzymatic activity. The enzymatic activity data obtained from the C209S mutant and IAA-modified wild-type enzymes indicate that Ag85 enzymes possessing small and moderate-sized polar residues have minimal enzymatic activity. The low activity of the C209G and C209A mutants show that Ag85 enzymes with small hydrophobic residues at position 209 will not afford high-level EBS resistance. The lack of activity in the C209F mutant suggests that large hydrophobic side chains cannot successfully replace cysteine. Further, as EBS covalently modifies all of the Mtb Ag85 mycolyltransferases at the same location and all three Ag85 enzymes possess the same native structure, it is logical to expect that mutations at the analogous C211 position of Ag85A and Ag85B will also profoundly affect the enzymatic activity of those enzymes. Combined with the initial inhibitory data of the Ag85C–EBS complex and further inspection of the Ag85C crystal structure near C209, the activity data from the Ag85C mutants suggest that structural features within the small, hydrophobic pocket that encompasses C209 in the native form of the enzyme cannot be maintained by an amino-acid side chain that differs from cysteine in either size or polarity. As the fbp genes that encode the enzymes of the Ag85 complex are likely synthetically lethal, the proposed mechanism of action suggests that compounds covalently modifying the conserved cysteine residue in enzymes of the Ag85 complex will forestall the selection of drug resistance through missense mutations. For example, if a C209S missense mutation in Ag85C prevents EBS from modifying the Ag85C–C209S mutant, the drug will still inactivate the Ag85A and Ag85B enzymes. Although the Ag85C–C209S mutant might retain 5–7% of its wild-type activity, such an organism would not be viable because neither Ag85A nor Ag85B would be functional. It is likely that this same result would occur for an analogous missense mutation in any of the fbp genes. In the extremely unlikely case of a coincident missense mutation in two or three of the fbp genes, EBS would not inhibit the mutant enzymes. However, it is likely that the very low level of enzymatic activity of the mutant Ag85 enzymes would be insufficient to promote bacterial viability or survival in the human host [26] . The primary question regarding the Ag85C–EBS crystal structure relates to the lack of observable density for any portion of the EBS molecule. This could be attributed to two different phenomena. First, structural disorder of EBS within the active site would decrease the observable density for the compound. When comparing the B-factors for the Sγ atom of C209 for the native Ag85C, Ag85C–DEP and Ag85C–EBS structures, it is clear that the C209 side chain is more dynamic in the Ag85C–EBS than in the other two structures. The average B-factors for the three structures are very similar (18.4–21.0 Å 2 ), as are the B-factors for the C209 Sγ atom in the native and Ag85C–DEP structure, which are 17 and 20 Å 2 , respectively. In contrast, the C209 Sγ atom of the Ag85C–EBS structure has a B-factor of 33 Å 2 and it is reasonable to expect the B-factor of a covalently attached selenium atom to be at least slightly higher than 33 Å 2 . The second phenomenon possibly contributing to the lack of EBS inhibitor density may result from performing the X-ray diffraction experiment. It is thoroughly documented that exposing protein crystals containing solvent-accessible disulphide bonds to ionizing radiation leads to sulphur oxidation and breaking of the associated disulphide bond [38] , [39] , [40] , [41] , [42] . As selenium oxidation in the context of a selenenylsulphide bond is more likely than sulphur oxidation in a disulphide bond, it can be expected that the selenenylsulphide bond between C209 and EBS is relatively labile during the X-ray diffraction experiment. Although either of these could lead to a decrease in the observable density for EBS, a combination of these two phenomena would further exacerbate the difficulty in observing density representing EBS in the active site. This new mode of inhibiting the enzymes of the Ag85 complex affords a novel approach for TB drug development that has not been previously considered, where covalent modification of active site-proximal residues disrupts the active site structure thereby forming an inactive enzyme. Although benzothiazinones inhibit the DprE1 epimerase by modifying a nonessential cysteine residue in the active site to prevent binding of substrate, resistance to those compounds develops in a facile manner through the mutation of the active site cysteine to a less reactive amino-acid residue [10] . As the cysteine has no role in the catalytic reaction carried out by DprE1, mutating this cysteine to either a serine or glycine promotes high-level resistance to benzothiazinones with the mutants retaining enzymatic activity [43] , [44] , [45] . Although EBS uses a similar chemical mechanism to inhibit Ag85C, the lack of activity observed for the C209 missense mutants indicates that high-level resistance to EBS is unlikely to occur. This hypothesis is further strengthened by analysis of sequence alignments of Ag85 homologues. The Mtb H37Rv genome encodes four Ag85 proteins (A–D) and other related esterases of unknown function [46] . As stated previously, Ag85A, B and C are known to possess mycolyltransferase activity, but Ag85D does not possess any mycolyltransferase activity [47] , [48] . It is intriguing that Ag85D has a serine residue at the site analogous to C209 in Ag85C and the X-ray crystal structure of Ag85D shows helix α9 to be in a relaxed conformation [48] . Furthermore, of the 76 Ag85-like sequences with a serine aligned to C209 of Ag85C, 67 (88%) are encoded by genes most closely related to the fbpD gene and therefore likely encode as enzymatically inactive Ag85D-like protein. When considering the potential of improving the MIC of EBS derivatives or inhibitors mimicking the EBS mechanism of action, the differences in rates of Ag85C modification observed for EBS and IAA suggest that efficacy of a novel Ag85 inhibitor using the described mechanism is more than simply a function of its ability to modify a conserved cysteine residue. Indeed, improvements can be made and efficacy will depend on properties of the inhibitor such as hydrophobicity, as the portion of the Ag85 active site harbouring C209 is almost exclusively hydrophobic. Also, it is reasonable to assume that the development of novel inhibitors with substantially improved affinity for regions of the Ag85 active site neighbouring C209 could lead to compounds with significantly improved inhibitory activity against the Ag85 complex and Mtb . The data described here offer the first look at the potent inhibition of the Mtb Ag85 complex by EBS, a compound that effectively inhibits the growth of drug-sensitive and drug-resistant strains, and its mechanism of action. Combined, these data show that covalently modifying C209 with EBS or other thiol reactive compounds is an excellent mechanism for inhibiting the Ag85 complex and any such compound will also significantly decrease the likelihood of developing drug resistance. Molecular cloning The molecular cloning of the segment of the Mtb fbpC encoding the secreted form of Ag85C included recombining the amplified gene with a pET29-based vector (EMD biosciences) using the NdeI and XhoI restriction sites, allowing a 6 × histidine tag at the C-terminus of the protein [33] . The genes encoding the secreted forms of Ag85A and Ag85B were placed between the NdeI and BamHI restriction sites of pET-28. For site-directed mutagenesis of Ag85C, the construct pET29- fbpC was used as a template to obtain the following mutants of Ag85C: C209A, C209S, C209G and C209F. The following primers, as well as their respective complements, purchased from Integrated DNA Technologies (IDT) were used for site-directed mutagenesis: 5′-CGGATCTGGGTGTAC GCC GGTAACGGCACACC-3′ (C209A), -5′-CGGATCTGGGTGTAC AGC GGTAACGGCACACCC-3′ (C209S), 5′-GGATCTGGGTGTAC GGC GGTAACGGCACA-3′ (C209G) and 5′-CCGGATCTGGGTGTAC TTC GGTAACGGCAC-3′ (C209F). The mutations were confirmed by nucleotide sequencing carried out by Eurofins MWG Operon. Protein purification of Ag85s and mutants For purification of the Ag85s and mutants, plasmids encoding the genes of interest were used to transform Escherichia coli T7 express cells (New England BioLabs). Bacterial cells were cultured at 37 °C in Luria Broth (Research Products International) supplemented with kanamycin (Gold Biotechnology) and chloramphenicol (Alfa Aesar). At OD 600nm 0.6, the temperature was decreased to 16 °C and protein expression was induced by addition of 1 mM isopropyl β- D -1-thiogalactopyranoside (Gold Biotechnology). The bacterial cells were harvested by centrifugation after 24- to 36-h induction and the pelleted cells were resuspended into 20 mM Tris pH 8.0, 25 mM imidazole and 5 mM β-mercaptoethanol (Nickel affinity binding buffer). Cell lysis was performed by addition of lysozyme (Sigma-Aldrich) and a sonication step (Sonicator 3000, Misonix). Then, nickel affinity and anion exchange purifications were carried out [33] . The protein was concentrated using ammonium sulphate precipitation (2.6 M). The precipitated protein was resuspended and dialyzed into either crystallization buffer (10 mM Tris pH 7.5, 2 mM EDTA and 1 mM DTT) or assay buffer (50 mM sodium phosphate pH 7.5, 1 mM DTT). The enzyme concentration was determined using absorbance spectroscopy at 280 nm. The ExPASy proteomics server, specifically the ProtParam function, was used to calculate the extinction coefficients of Ag85C and its different mutants [49] . Recombinant Mtb Ag85A and B were purified using the same protocol. Ag85C fluorometric assay The fluorescent compound resorufin butyrate (Santa Cruz Biotechnology) was used as an acyl donor whereas trehalose was used as an acyl acceptor. Stock solutions of resorufin butyrate were prepared in DMSO and diluted 100-fold in each reaction. Trehalose was dissolved in 50 mM sodium phosphate (pH 7.5) buffer in which all the reactions were performed. Kinetic parameters of resorufin butyrate were determined by fluorescence using λ exc =500 nm and λ em =593 nm. The reactions were carried out at 37 °C on a Synergy H4 Hybrid Reader (BioTek). The concentration of trehalose was fixed at 4 mM while resorufin butyrate concentrations were varied from 0 to 125 μM. Ag85C was used at a concentration of 500 nM. Reactions performed in triplicate were initiated by addition of resorufin butyrate. Non-linear regression analysis of kinetic data was carried out using Prism 5 software. To determine the Z , value [30] , a set of 24 positive controls containing 500 nM Ag85C and 24 negative controls lacking Ag85C were carried out using fixed resorufin butyrate concentration of 100 μM. A Z , value of 0.82 was obtained. The NIH clinical collection was screened using the same conditions as above. The activities of the different mutants as well as the samples used for mass spectrometry were assayed using an enzyme concentration of 500 nM and conditions identical to those used for the Z , determination and screening. The alkylation reactions were carried out using concentrations of IAA (Sigma) between 2.6 and 51.2 mM. The sample activities were tested as above after 1- and 24-h incubation and compared each time with a sample of Ag85C without IAA. Ag85C activity assays were performed as mentioned above. Time course experiment was also carried out as mentioned above using 5 μM EBS. In vitro TMM transferase and in vivo assays Growth conditions: Mtb mc 2 6206 (ΔPanCD ΔLeuCD) was grown in Middlebrook 7H9-OADC medium supplemented with 0.05% Tween 80, 0.2% casaminoacids, 0.0048% pantothenate and L -Leucine (50 μg ml −1 ). MIC determination The MIC values of EBS against Mtb H37Rv strain mc 2 6206 was determined in 7H9-OADC–Tween 80 broth supplemented with 0.5% glycerol, 0.2% casaminoacids, 0.0048% pantothenate and 50 μg ml −1 L -Leucine in 96-well microtiter plates using the colorimetric resazurin microtiter assay. Growth was measured by visual readout. Whole-cell radiolabeling experiments Radiolabeling of whole mycobacterial cells with [1,2- 14 C]-acetic acid (0.5 μCi ml −1 ; specific activity, 57 Ci mol −1 ; NEN Radiochemicals) was performed for 16 h with shaking. The radiochemical was added to the cultures at the same time as the inhibitor. Analytical procedures Total lipid extraction from bacterial cells and preparation of mycolic acid methyl esters from delipidated cells followed standard procedures [36] , [50] . Lipids and mycolic acid methyl esters were analysed by TLC (chloroform:methanol:water; 20:4:0.5, v/v for lipids and n -hexanes:ethyl acetate; 95:5, v/v for mycolic acid methyl esters) on aluminum-backed silica gel 60-precoated plates F254 (Merck). Radiolabeled products were visualized by exposing the TLC plates to Kodak X-Omat AR films at −80 °C and were quantified using a PhosphorImager (Typhoon, GE Healthcare). Mycolyltransferase assays A TMM transesterification assay was used to determine the mycolyltransferase activity of purified Ag85A, B, and C. Briefly, the activity of the Ag85 proteins (8 μM) was measured in the presence of cold TMM purified from Mtb (15 μg), [U- 14 C]-trehalose (1.25 μCi ml −1 ; specific activity, 600 mCi mol −1 ; American Radiolabeled Chemicals) and 0 or 10 μM EBS. Assays were conducted in a total volume of 200 μl and allowed to proceed for 60 min at 37 °C. The reaction was stopped by adding 3 ml of CHCl 3 :CH 3 OH (2:1) and 300 μl of water. The organic extractable material containing the glycolipid products of the reaction was analysed by TLC (chloroform:methanol:water; 20:4:0.5, v/v) as described in analytical procedures and revealed by autoradiography. The same volume of sample was loaded in each lane. The amount of radioactivity incorporated in the products of interest was semiquantified using a Phosphorimager. Mass spectrometry The protein samples were buffer exchanged against 10 mM ammonium acetate pH 7.0 and concentrated to 0.5 mg ml −1 using a 3 kDa ultracentrifugation device (Millipore). EBS from a 10 mM stock in DMSO was mixed at a final concentration of 200 μM with protein samples. A control reaction used just DMSO to a final concentration of 2% DMSO. The samples were incubated for 2 h on ice. The samples were then buffer exchanged three times with 10 mM ammonium acetate pH 7.0 to remove any DMSO and excess EBS. Half of the sample containing 200 μM of EBS was treated with 1 mM DTT and incubated for another hour. The samples were diluted in acetonitrile/water (1:1, v/v) containing 0.1% formic acid to a protein concentration of 0.1 mg ml −1 and analysed on an ESI Q-TOF Micro mass spectrometer (Waters) in positive ion mode. ESI-MS data were acquired and analysed by MassLynx software (Waters). The alkylation reaction was performed using 38 mM of IAA. In-solution trypsin digestion of the different protein complexes was also performed with a standard protocol using sequencing-grade trypsin (Promega). Peptide mass determination was carried out on a MALDI-TOF/TOF mass spectrometer (Bruker Daltonics). Crystallization Crystals of the Ag85 (5 mg ml −1 ) in the presence of EBS, and Ag85C–C209S (5 mg ml −1 ) were grown using hanging-drop vapour diffusion. Ag85C–C209S was crystallized in 0.1 M bis-tris pH 6.5, 25% w/v polyethylene glycol 3350 whereas wild-type Ag85C was co-crystallized in the presence of 200 μM EBS dissolved in DMSO (final concentration DMSO: 2%) in 25% w/v polyethylene glycol 1500 (Hampton Research). For the Ag85C–EBS and Ag85C–C209S proteins, crystals formed after 1 month. All crystals were flash-cooled in liquid nitrogen prior to data collection. Diffraction data were collected at the LS-CAT beamline at the Advance Photon Source Argonne National Laboratory (APS-ANL, IL), at wavelengths of 0.97922 and 0.97856 Å for the Ag85C–EBS and Ag85–C209S structures, respectively. Structure determination Diffraction data were indexed, integrated and scaled using HKL2000 [51] . EPMR (Evolutionary Program for Molecular Replacement) was used to perform the molecular replacement for each data set using PDB 1DQZ (Ag85C WT [23] ) as a model. Rigid body refinement, simulated annealing, positional and B-factor refinement was carried out using PHENIX [52] . Manual refinement was performed using COOT [53] . The final refined model results in a Ramachandran plot with 97.0% of residues in the favored region and 3.0% in the allowed for the Ag85C–EBS structure. In the Ag85C–C209S structure, the favored and allowed values are 97.5 and 2.1%, respectively. Accession codes: The atomic coordinates of novel structures have been deposited in the Protein Data Bank with accession codes 4MQL , 4MQM . How to cite this article: Favrot, L. et al . Mechanism of inhibition of Mycobacterium tuberculosis antigen 85 by ebselen. Nat. Commun. 4:2748 doi: 10.1038/ncomms3748 (2013).